Use of the CRISPR/Cas9 system as an intracellular defense against HIV-1 infection in human cells To combat hostile viruses, bacteria and archaea have evolved a unique antiviral defense system composed of clustered regularly interspaced short palindromic repeats (CRISPRs), together with CRISPR-associated genes (Cas). The CRISPR/Cas9 system develops an adaptive immune resistance to foreign plasmids and viruses by creating site-specific DNA double-stranded breaks (DSBs). Here we adapt the CRISPR/Cas9 system to human cells for intracellular defense against foreign DNA and viruses. Using HIV-1 infection as a model, our results demonstrate that the CRISPR/Cas9 system disrupts latently integrated viral genome and provides long-term adaptive defense against new viral infection, expression and replication in human cells. We show that engineered human-induced pluripotent stem cells stably expressing HIV-targeted CRISPR/Cas9 can be efficiently differentiated into HIV reservoir cell types and maintain their resistance to HIV-1 challenge. These results unveil the potential of the CRISPR/Cas9 system as a new therapeutic strategy against viral infections. Viral infections underlie a variety of different human diseases, including life-threatening AIDS [1] . Currently, treatment for such diseases focuses on drugs and vaccines that specifically target the viral proteins or inhibit host–viral interactions [2] , [3] . However, the nature of lentiviral infections, whereby the virus, such as human immunodeficiency virus (HIV), invades immune cells and integrates into the host genome to establish its latent infection, has created a huge obstacle with respect to developing efficient vaccines [4] , [5] . These lentiviral features and the lack of immune response to eliminate the latent viral genome from reservoirs constitute the major challenges that need to be overcome, to develop efficient therapies [6] , [7] , [8] . The clustered regularly interspaced short palindromic repeat (CRISPR)/Cas9 system is known to play a major role in the adaptive immune response to foreign plasmids and viruses in about 40% of bacteria [9] , [10] , [11] . Recently, several research groups have successfully applied the type II CRISPR system—SpCas9 protein from Streptococcus pyogenes with guided RNA (gRNA)—for targeted genome editing in diverse cell types and organisms, including human cells [12] , [13] , [14] . Most recently, a couple of studies have demonstrated the excision of the HIV-1 provirus from the host cell genome using gene-editing tools [15] , [16] , [17] , [18] . Here we apply the CRISPR/Cas9 system to directly target and disrupt the reverse-transcribed products of the lentiviral RNA genome during their life cycle within host cells. We screen multiple potential gRNA target sites in the HIV genome and identify optimized targets that enable effective and long-term protection against HIV-1 infection in primary human T cells and human pluripotent stem cell (hPSC)-derived HIV reservoir cell types. The strategy presented here may open a new avenue for research and novel clinical strategies against viral infectious diseases. On early entry into their target cells, lentiviruses reverse transcribe their single-stranded RNA genome into double-stranded DNA (dsDNA) by a virally encoded reverse transcriptase [19] . The resulting viral DNA is then transported into the cell nucleus and integrated into the host genome as a latent provirus, thereby avoiding detection from the host’s immune system [8] . During these early events in the viral life cycle, the lentivirus is released from its capsid ( Fig. 1a ). We hypothesized that this exposed virus genome would be susceptible to targeted disruption by sequence-specific DNA nucleases inside the host cells. To test this, we first used replication-incompetent pseudotyped lentiviruses as the target to restrict our analysis to a single round of viral infection. Target gRNAs were designed against the enhanced green fluorescent protein (EGFP) coding region as well as the non-coding long terminal repeat (LTR) of an EGFP reporter lentivirus ( Fig. 1b ). These gRNAs were designed to only target the sequences unique to the viral reporter and not present in the human genome. To directly monitor Cas9 nuclease expression inside cells, we first constructed a human codon-optimized Cas9-2A-mCherry reporter (hCas9-mCh), which has been confirmed to be functionally equivalent to the wild-type hCas9 in an EGFP reporter rescue assay similar to a previously reported one [20] ( Supplementary Fig. 1a ). Therefore, the expression of hCas9 can be tracked by the mCherry signal. 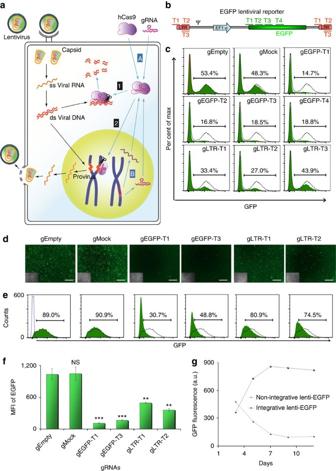Figure 1: CRISPR/Cas9 directed disruption of lentivirus infection. (a) Model of CRISPR/Cas9 directed intracellular defense against lentiviral infection. hCas9 and its gRNA can be synthesized from either transfected plasmids (module A) or knockin expression cassettes (module B). After synthesis, hCas9 and gRNA assemble and work as an antiviral module in different steps. Once penetrating into the host cells, virally encoded reverse transcriptase uses the lentiviral RNA genome as a template for the synthesis of viral cDNA. Viral integrase binds and processes the LTR and assists in the insertion of the viral cDNA into the host genome. During these processes, the viral genome is unprotected by its envelope and capsid, rendering the viral cDNA vulnerable to cleavage by DNA endonucleases. In our study, the CRISPR/Cas9 system was adapted for human cells as an antiviral module, which bound and disrupted the viral genome of both pre-integration viral DNA (Step 1) and integrated provirus (Step 2). (b) Seven gRNAs were designed and used with hCas9 to target corresponding regions in the EGFP reporter lentivirus, including gEGFP-T1 to -T4 and gLTR-T1 to -T3. (c) FACS analysis of HEK293 cells that were pretreated with hCas9-mCh and gRNAs for 20∼24 h, and then challenged by EGFP reporter lentiviruses for 4 days. gEmpty is an empty gRNA vector and gMock (as the gS35 inSupplementary Fig. 1) is a non-targeting mock gRNA. (d–g) The CRISPR/Cas9 system can direct targeted disruption of the non-integrative lentivirus. (d) Fluorescence microscopy images of HEK293 cells pretreated with CRISPR/Cas9 followed by non-integrative lentivirus infection for 3 days. Insets show bright field images. Scale bar, 500 μm. (e) EGFP expressions of invading non-integrated lentivirus were measured by flow-cytometric analysis. Overlay histogram depicts the gEmpty in the first panel and the dashed blue line indicates the non-treatment cells. (f) The bar graph represents the average of MFI (mean fluorescence intensity) from triplicates of FACS analysis. Statistical analysis determined using unpairedt-test (***P<0.001; **P<0.01) (g) Time-course analysis of EGFP expression from integrative and non-integrative lentiviruses without any treatment with CRISPR/Cas9. The results showed that the integrative lenti-EGFP expressed constitutively from 7 days after infection, whereas the expression of non-integrative lenti-EGFP gradually reduced over time. Figure 1: CRISPR/Cas9 directed disruption of lentivirus infection. ( a ) Model of CRISPR/Cas9 directed intracellular defense against lentiviral infection. hCas9 and its gRNA can be synthesized from either transfected plasmids (module A) or knockin expression cassettes (module B). After synthesis, hCas9 and gRNA assemble and work as an antiviral module in different steps. Once penetrating into the host cells, virally encoded reverse transcriptase uses the lentiviral RNA genome as a template for the synthesis of viral cDNA. Viral integrase binds and processes the LTR and assists in the insertion of the viral cDNA into the host genome. During these processes, the viral genome is unprotected by its envelope and capsid, rendering the viral cDNA vulnerable to cleavage by DNA endonucleases. In our study, the CRISPR/Cas9 system was adapted for human cells as an antiviral module, which bound and disrupted the viral genome of both pre-integration viral DNA (Step 1) and integrated provirus (Step 2). ( b ) Seven gRNAs were designed and used with hCas9 to target corresponding regions in the EGFP reporter lentivirus, including gEGFP-T1 to -T4 and gLTR-T1 to -T3. ( c ) FACS analysis of HEK293 cells that were pretreated with hCas9-mCh and gRNAs for 20 ∼ 24 h, and then challenged by EGFP reporter lentiviruses for 4 days. gEmpty is an empty gRNA vector and gMock (as the gS35 in Supplementary Fig. 1 ) is a non-targeting mock gRNA. ( d – g ) The CRISPR/Cas9 system can direct targeted disruption of the non-integrative lentivirus. ( d ) Fluorescence microscopy images of HEK293 cells pretreated with CRISPR/Cas9 followed by non-integrative lentivirus infection for 3 days. Insets show bright field images. Scale bar, 500 μm. ( e ) EGFP expressions of invading non-integrated lentivirus were measured by flow-cytometric analysis. Overlay histogram depicts the gEmpty in the first panel and the dashed blue line indicates the non-treatment cells. ( f ) The bar graph represents the average of MFI (mean fluorescence intensity) from triplicates of FACS analysis. Statistical analysis determined using unpaired t -test (*** P <0.001; ** P <0.01) ( g ) Time-course analysis of EGFP expression from integrative and non-integrative lentiviruses without any treatment with CRISPR/Cas9. The results showed that the integrative lenti-EGFP expressed constitutively from 7 days after infection, whereas the expression of non-integrative lenti-EGFP gradually reduced over time. Full size image These gRNAs, together with hCas9, caused a significant reduction in the percentage of cells counted as GFP positive as well as in GFP fluorescence intensity in infected cells. The reduction ranged from 18% to 72%, depending on the target sites of gRNA ( Fig. 1c , Supplementary Fig. 1d,f,h and Supplementary Tables 1 and 2 ). Meanwhile, pretreatment with either hCas9 or gRNA individually did not result in any disruption of EGFP expression from viruses ( Supplementary Fig. 1b,c ), indicating that neither hCas9 nor gRNA individually inhibits viral gene expression without specific targeting. We further examined the antiviral target specificity by comparing CRISPR/Cas9-mediated disruption of different lentiviruses (lentivirus that has either EGFP or mCherry coding sequence within the same backbone; Supplementary Fig. 2a,b ). By targeting different regions, our results indicate that Cas9, guided by different gRNAs, accurately distinguishes between these two lentiviral vectors. Our data suggest two possible mechanisms for the Cas9-mediated inactivation of viral gene expression. First, Cas9 could directly target the viral genomic DNA, when the virus enters the cell and reverse transcribes into dsDNA before integration into the host genome ( Fig. 1a , step 1). Second, Cas9 could disrupt the proviral elements already integrated in the host genome ( Fig. 1a , step 2). To distinguish between these possibilities, we repeated the above-mentioned experiment with a non-integrative EGFP lentivirus as the target. Intriguingly, our results show that Cas9 inactivates viral EGFP expression to a similar extent regardless of the integration status of the lentivirus ( Fig. 1d–g ). Moreover, instead of integrating into the host genome, lentiviruses can transiently present in a circular double-stranded format in the host cells. The CRISPR/CRISPR-associated genes (Cas) system has been reported to functionally inactivate invading plasmids in bacterial cells [10] ; we therefore examined whether the CRISPR/Cas9 system can also be used to inactivate circular foreign plasmids (double-stranded circular DNA) in human cells. By using the same backbone of EGFP reporter in previous lentivirus assays ( Supplementary Fig. 1d,f,h ), the CRISPR/Cas9 system showed its ability to inactivate the expression of invading plasmids at a comparable level, to disrupt the infectious lentivirus ( Supplementary Fig. 1e,g,i ). Disruption/eradication of integrated proviral genome To further examine whether the proviral genome of lentivirues can be disrupted or eradicated from the human genome by the CRISPR/Cas9 system, we established several stable HEK293 cell lines bearing different numbers of integrated proviruses. After transfection of CRISPR/Cas9 into these cells, the fluorescent signal from the virally expressed GFP gradually reduced and finally reached the same level as that of the uninfected negative control cells ( Fig. 2a,f ). The time-course results shown here also indicate that although expressed transiently, CRISPR/Cas9 can mediate permanent inhibition of viral expression due to disruption of proviruses at the DNA level, which is different than the transient repression of viral expression by other methods, such as RNA interference [21] , [22] , [23] . Meanwhile, the molecular analysis showed that the disruption of GFP expression was caused by either insertion/deletion or full-length excision ( Fig. 2b–e ). Our result also showed that the CRISPR/Cas9 system could efficiently disrupt the activity of proviruses regardless of copy numbers ( Fig. 2b,d ). This effect was also contingent on target gRNA specificity, as we showed by using different gRNAs to differentially target either EGFP or mCherry proviruses ( Supplementary Fig. 2c,d ). In addition, after a secondary delivery of the CRISPR/Cas9 system, the levels of viral expression were further decreased, suggesting that a potential low-dose chronic treatment regiment, which may be less cytotoxic, could be effective in eradicating proviruses over time ( Fig. 2g ). In summary, these results indicate that the CRISPR/Cas9 system can mediate targeted disruption of both pre-integration viruses and integrated proviruses with dsDNA in either linear or circular format. More comprehensive mechanisms of CRISPR/Cas system-mediated foreign DNA disruption in both bacterial and human cells remain to be further studied. 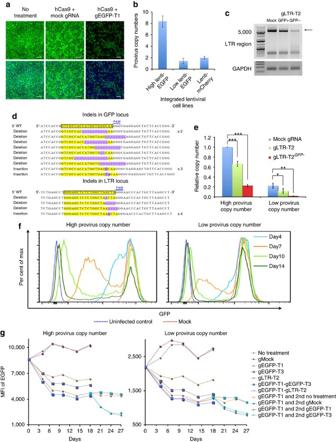Figure 2: CRISPR/Cas9 directed disruption of integrated lentivirus. CRISPR/Cas9-mediated disruption of integrated lenti-proviral DNA in infected HEK293 cells. (a) Top: confocal images of cells with high copy numbers of EGFP proviral DNA that were co-transfected with hCas9 and either gEGFP-T1 (right panels) or mock gRNA (middle panels). Left panels show untreated cells. Images were taken at 14 days after transfection. Bottom: confocal images with DAPI staining (blue). Scale bars, 50 μm. (b) Determination of provirus copy numbers in three different lentiviral integrated HEK293 cell lines. (c) PCR analysis of proviral DNA. The amount of full-length provirus (arrow) was reduced in the GFP-negative cells generated by CRISPR/Cas9-mediated lentiviral disruption. (d) DNA sequencing analysis of the CRISPR/Cas9 target sites in the EGFP proviruses. Two examples shown here were treated with hCas9 and either gEGFP-T1 (top) or gLTR-T2 (bottom). Sequences identified multiple times were marked accordingly on the right. (e) Proviral copy number quantitation by qPCR. Statistical analysis determined using unpairedt-test (***P<0.001; **P<0.01; *P<0.1). (f) FACS analysis of proviral EGFP expression at different days after transfection of hCas9 and gRNAs into cells with either high or low provirus copy numbers as determined inb. (g) FACS analysis of EGFP expression at different days after treatment of the integrated lenti-EGFP HEK293 cell lines with hCas9-mCh and the corresponding gRNA. CRISPR/Cas-mediated disruption of integrated lentiviral DNA can be augmented by either multiplexed site-directed targeting or combinatorial treatments. gEGFP-T1-gEGFP-T3 and gEGFP-T1-gLTR-T2 represent multiplexed targeting. In addition, to examine the effects of multiple treatments, we introduced secondary transfection of hCas9 together with the indicated gRNAs into provirus Lenti-EGFP cells that were pre-treated with hCas9-gEGFP-T1 for 18 days. Figure 2: CRISPR/Cas9 directed disruption of integrated lentivirus. CRISPR/Cas9-mediated disruption of integrated lenti-proviral DNA in infected HEK293 cells. ( a ) Top: confocal images of cells with high copy numbers of EGFP proviral DNA that were co-transfected with hCas9 and either gEGFP-T1 (right panels) or mock gRNA (middle panels). Left panels show untreated cells. Images were taken at 14 days after transfection. Bottom: confocal images with DAPI staining (blue). Scale bars, 50 μm. ( b ) Determination of provirus copy numbers in three different lentiviral integrated HEK293 cell lines. ( c ) PCR analysis of proviral DNA. The amount of full-length provirus (arrow) was reduced in the GFP-negative cells generated by CRISPR/Cas9-mediated lentiviral disruption. ( d ) DNA sequencing analysis of the CRISPR/Cas9 target sites in the EGFP proviruses. Two examples shown here were treated with hCas9 and either gEGFP-T1 (top) or gLTR-T2 (bottom). Sequences identified multiple times were marked accordingly on the right. ( e ) Proviral copy number quantitation by qPCR. Statistical analysis determined using unpaired t -test (*** P <0.001; ** P <0.01; * P <0.1). ( f ) FACS analysis of proviral EGFP expression at different days after transfection of hCas9 and gRNAs into cells with either high or low provirus copy numbers as determined in b . ( g ) FACS analysis of EGFP expression at different days after treatment of the integrated lenti-EGFP HEK293 cell lines with hCas9-mCh and the corresponding gRNA. CRISPR/Cas-mediated disruption of integrated lentiviral DNA can be augmented by either multiplexed site-directed targeting or combinatorial treatments. gEGFP-T1-gEGFP-T3 and gEGFP-T1-gLTR-T2 represent multiplexed targeting. In addition, to examine the effects of multiple treatments, we introduced secondary transfection of hCas9 together with the indicated gRNAs into provirus Lenti-EGFP cells that were pre-treated with hCas9-gEGFP-T1 for 18 days. Full size image Targeting site screening against HIV-1 genome As there can be important differences between how viral vectors, wild-type and wild-type-like viruses infect cells, we tested whether the CRISPR/Cas9 system can disrupt the generic HIV-1 viral genome during viral infection. After filtering out sequences with high homology to the human genome (see Methods), we selected and screened multiple gRNA-targeting sites within the HIV-1 genome, including the structural ( gag and env ), enzymatic ( pol ) and accessory genes ( vif and rev ), as well as LTRs ( Fig. 3a and Supplementary Table 2 ). The GFP expression levels of VSV.G-HIV-1 NL4-3-ΔE-GFP in the cells that were treated with HIV-specific gRNA and hCas9 were 48% ∼ 92% lower than the cells transfected with empty gRNA vector. However, this reduction did not occur when we used mock gRNA with hCas9 ( Fig. 3b ). We also noted that gRNAs targeting LTR sequences (especially the R region) were more effective than others, indicating the importance of the LTR-R region in HIV expression. 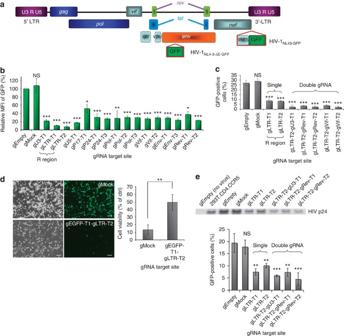Figure 3: CRISPR/Cas9-directed disruption of HIV-1 virus. (a) HIV virus constructs used to generate the pseudotyped (HIV-1NL4-3-ΔE-GFP) and wild-type reporter virus (HIV-1NL43-GFP) for infection in this study. (b) FACS analysis of the average of MFI (mean fluorescence intensity) of EGFP in HIV-1NL4-3-ΔE-GFPinfected HEK293 cells transfected with hCas9 together with a variety of gRNAs against the HIV genome. SeeSupplementary Table 1for details about the gRNAs. (c) Comparison of antiviral disruption with single or double gRNAs performed in 293T.CD4.CCR5 cells infected with HIV-1NL4-3-ΔE-GFP. (d) Cell viability analysis of cells containing CRISPR/Cas9 following HIV-1 infection. Bright-field and fluorescent images show that gEGFP-T1-gLTR-T2 HEK293 cells are resistant to HIV-1NL4-3-ΔE-GFPinfection and have higher cell viability (bottom panels on the left and graph on the right) when compared with gMock treated cells (top panels). Scale bars, 100 μm. (e) CRISPR/Cas9-mediated antiviral activity against wild-type HIV-1 reporter virus (HIV-1NL43-GFP) was monitored by the levels of the viral p24 protein (top) and GFP reporter expression (bottom). All statistical comparisons were made by unpairedt-test (***P<0.001; **P<0.01; *P<0.1; NS, no significant) with at least three replicates. Figure 3: CRISPR/Cas9-directed disruption of HIV-1 virus. ( a ) HIV virus constructs used to generate the pseudotyped (HIV-1 NL4-3-ΔE-GFP ) and wild-type reporter virus (HIV-1 NL43-GFP ) for infection in this study. ( b ) FACS analysis of the average of MFI (mean fluorescence intensity) of EGFP in HIV-1 NL4-3-ΔE-GFP infected HEK293 cells transfected with hCas9 together with a variety of gRNAs against the HIV genome. See Supplementary Table 1 for details about the gRNAs. ( c ) Comparison of antiviral disruption with single or double gRNAs performed in 293T.CD4.CCR5 cells infected with HIV-1 NL4-3-ΔE-GFP . ( d ) Cell viability analysis of cells containing CRISPR/Cas9 following HIV-1 infection. Bright-field and fluorescent images show that gEGFP-T1-gLTR-T2 HEK293 cells are resistant to HIV-1 NL4-3-ΔE-GFP infection and have higher cell viability (bottom panels on the left and graph on the right) when compared with gMock treated cells (top panels). Scale bars, 100 μm. ( e ) CRISPR/Cas9-mediated antiviral activity against wild-type HIV-1 reporter virus (HIV-1 NL43-GFP ) was monitored by the levels of the viral p24 protein (top) and GFP reporter expression (bottom). All statistical comparisons were made by unpaired t -test (*** P <0.001; ** P <0.01; * P <0.1; NS, no significant) with at least three replicates. Full size image Next, we examined the CRISPR/Cas9 antiviral system in latently infected T-cell lines containing a full-length integrated HIV genome. The A2 and 10.6 J-lat clones contain a GFP open reading frame in place of the nef gene and a frameshift mutation in the env gene [24] . The latent viral load was greatly reduced by co-transfection of Cas9 and anti-LTR gRNAs, as evidenced by a six- to sevenfold reduction in viral GFP reactivation by Phorbol 12-myristate 13-acetate (PMA) and Tumor-necrosis factor-alpha (TNF-alpha) ( Supplementary Fig. 3a ). The GFP reduction correlated with the disruption of the viral genome in the targeting regions ( Supplementary Fig. 3b ). Multiplexed targeting of HIV-1 genome by CRISPR/Cas9 In microbial CRISPR systems, when a plasmid or virus enters the bacterial host, fragments of the foreign DNA can be seized as ‘spacers’ and assembled with identical ‘repeats’ to form tandem arrays that become the templates for multiplexed foreign DNA targeting [11] , [25] . This led us to think that the ability of the CRISPR/Cas system to perform multiplexed genome engineering is a major strength that could be leveraged to develop an antiviral method in human cells. Thus, we next examined multiplexed disruption of viral infection by co-delivery of hCas9 and multiple gRNAs. As the results show in Fig. 3c , the multiplex CRISPR/Cas9 system abated the infectious virus or proviral genome inside the host cells more completely when compared with the singly targeted Cas9. Meanwhile, cell viability also increased with the multiplex CRISPR/Cas9 system, which is consistent with more effective elimination of the toxic infectious virus ( Fig. 3d ). We further examined the CRISPR/Cas9-mediated protection against infectious wild-type HIV, HIV-1 NL43-GFP , which recapitulates the early and late events in the viral life cycle, including production of viral RNAs and release of virions from host cells. Both the release of p24 viral protein and production of GFP were decreased, compared with controls, especially in the double gRNA systems ( Fig. 3e ). This suggests that the multiplex CRISPR/Cas9 system is highly effective in suppressing wild-type HIV replication and reactivation in human cells. Stable expression of Cas9 against HIV-1 in physiological cells To test the possibility of conferring intracellular immunity against lentiviral infections using the CRISPR/Cas9 system, we constructed several Cas9/gRNA stable cell lines by using piggyBac (PB) transposon-mediated genome engineering systems. Our results show that these stable lines are sufficiently protected against subsequent viral infections ( Supplementary Fig. 3c–g ). The level of antiviral protection conferred by stably integrated Cas9/gRNA was sufficient to inactivate the lentiviral expression in a similar manner to those obtained by transient transfection ( Fig. 1 ). To further investigate whether the CRISPR/Cas9 system can immunize cells against replicated wild-type HIV-1 over a longer period of time, we tracked viral infectivity in a human T-cell line for 14 days. Sup-T1 cells with stably integrated Cas9 and gRNA targeting a variety of HIV-1 genome sequences were infected with HIV-1 NL43-GFP ( Fig. 4a ). Although the infection of HIV-1 increased over time in the control gRNA group, the groups with HIV-1-targeted gRNAs effectively reduced the level of viral expression. In particular, the groups with combinations of gRNAs targeting the U3 and R regions of the HIV-1 LTR maintained a low level of viral expression even over 14 days of HIV-1 infection, although most host cells had been infected and had a poor survival rate in the no CRISPR treatment control population ( Fig. 4b ). This prolonged inhibition of viral expression is consistent with a disruption of viral replication in multiple cycles of viral infection. To demonstrate the disruption of HIV infection in a more physiological context, we applied the CRISPR/Cas9 antiviral system to human primary CD4+ T cells. Using more than five independent T-cell donors, our results showed that CRISPR/Cas9 targeting HIV-1 LTR R regions efficiently reduced virus production by more than threefold compared with the controls ( Fig. 4c ). 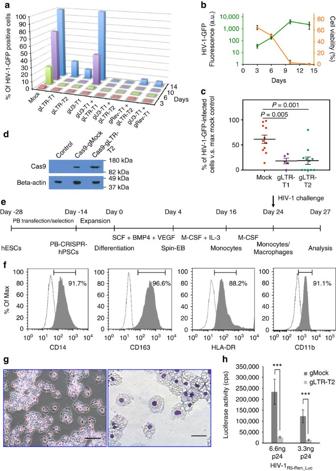Figure 4: Prevention of wild-type HIV-1 virus infection in physiological cell types by the CRISPR/Cas9 system. (a) Time-course analysis of HIV-1NL43-GFPinfection in Sup-T1 cells that stably express hCas9 and diverse gRNAs against HIV-1. The percentage of HIV-1 infection was measured by the percentage of GFP expression cells after 3, 6, 10 and 14 days HIV-1NL43-GFPvirus infection. (b) The kinetics of viral replication and infected cell viability of HIV-1NL43-GFPvirus in Sup-T1 cells. (c) hCas9 co-treated with guide RNA against LTR-R regions showed reduction of HIV-1NL43-GFPexpression in human primary T cells after 3 days HIV-1 infections. Each dot represents the percentage of GFP-positive cell number from an individual sample with normalization by the GFP cell percentage of maximum mock gRNA control. (d) Western blotting analysis of Cas9 protein expression in the hPSCs by the monoclonal anti-Cas9 antibody. (e) Schematic experimental procedures for the generation of PB-CRISPR/Cas9-hPSCs and differentiation of monocytes/macrophages lineages for the HIV-1 challenge assays. (f) FACS analysis of PB-CRISPR/Cas9-hPSCs-derived monocytes/macrophages. (g) Eosin–methylene blue staining of PB-CRISPR/Cas9-hPSCs-derived monocytes/macrophages spun on slides. Scale bars, 100 μm (left) and 50 μm (right). (h) Luciferase analysis of PB-CRISPR/Cas9-hPSCs-derived monocytes/macrophages containing either gMock or gLTR-T2 at 3 days after infection of HIV-1R5-Ren_Luc. Means were compared by unpairedt-test (***P<0.001). Figure 4: Prevention of wild-type HIV-1 virus infection in physiological cell types by the CRISPR/Cas9 system. ( a ) Time-course analysis of HIV-1 NL43-GFP infection in Sup-T1 cells that stably express hCas9 and diverse gRNAs against HIV-1. The percentage of HIV-1 infection was measured by the percentage of GFP expression cells after 3, 6, 10 and 14 days HIV-1 NL43-GFP virus infection. ( b ) The kinetics of viral replication and infected cell viability of HIV-1 NL43-GFP virus in Sup-T1 cells. ( c ) hCas9 co-treated with guide RNA against LTR-R regions showed reduction of HIV-1 NL43-GFP expression in human primary T cells after 3 days HIV-1 infections. Each dot represents the percentage of GFP-positive cell number from an individual sample with normalization by the GFP cell percentage of maximum mock gRNA control. ( d ) Western blotting analysis of Cas9 protein expression in the hPSCs by the monoclonal anti-Cas9 antibody. ( e ) Schematic experimental procedures for the generation of PB-CRISPR/Cas9-hPSCs and differentiation of monocytes/macrophages lineages for the HIV-1 challenge assays. ( f ) FACS analysis of PB-CRISPR/Cas9-hPSCs-derived monocytes/macrophages. ( g ) Eosin–methylene blue staining of PB-CRISPR/Cas9-hPSCs-derived monocytes/macrophages spun on slides. Scale bars, 100 μm (left) and 50 μm (right). ( h ) Luciferase analysis of PB-CRISPR/Cas9-hPSCs-derived monocytes/macrophages containing either gMock or gLTR-T2 at 3 days after infection of HIV-1 R5-Ren_Luc . Means were compared by unpaired t -test (*** P <0.001). Full size image To test whether the CRISPR/Cas9 system could confer HIV-1 resistance to haematopoietic lineages that could serve as latent HIV reservoirs, such as monocyte/macrophage lineages [26] , several piggyBac -mediated anti-HIV-1 hPSC lines were generated and confirmed for Cas9 protein expression by western blotting ( Fig. 4d ). These CRISPR/Cas9-hPSCs can be differentiated into monocytes/macrophages using a feeder-free protocol [27] , [28] ( Fig. 4e ). A relatively homogenous population of monocytes/macrophages was efficiently differentiated from the PB-CRISPR/Cas9 hPSCs ( Fig. 4f,g ). The differentiated cells were inoculated with an M-tropic virus clone, HIV-1 R5-Ren_Luc , for 3 days before the analysis ( Fig. 4h ). The results show that engineered hPSCs can confer resistance to HIV-1 infection in derived monocytes/macrophages. The fact that PB-CRISPR/Cas9 hPSCs could be stably maintained for multiple passages and efficiently differentiated suggests that the HIV-1-targeted CRISPR/Cas9 system does not have overt genotoxicity. To further study this point, we evaluated the off-target effect of the PB-CRISPR/Cas9 hPSCs against the most efficient LTR-T2 target region. From the analysis of the top five off-target candidates with high sequence similarity in the exonic regions of the human genome, there was no significant off-target effect in any of the analysed clones of hPSCs ( Supplementary Table 3 ). Meanwhile, there was no detectable off-target effect in the PB-CRISPR/Cas9 HEK293 cells when we examined the top five off-target candidates with high sequence homology to either gLTR-T1 or gLTR-T2 in these lines ( Supplementary Table 3 ). Antiviral activities against retrovirus and adenovirus To test the generality of the CRISPR/Cas9-mediated antiviral immunity in human cells, we used retrovirus as well as adenovirus, which have a dsDNA genome, as virus targets. Consequently, the expression of retrovirus and adenovirus was significantly decreased by the CRISPR/Cas9 system, suggesting a broad application in antiviral therapies ( Supplementary Fig. 4a–j ). Meanwhile, the CRISPR/Cas9 system has been applied to target other infective viruses, such as papillomavirus, type I herpes simplex virus and hepatitis B virus by other groups [26] , [29] , [30] . These results demonstrated the generality of the CRISPR/Cas9 system for application as either a viral genome editing tool or anti-viral treatment. Finally, we examined whether the inactivated form of Cas9 fused with a transcriptional repressor, KRAB domain (dCas9-KRAB), could also repress HIV-1 expression in mammalian cells. Without the generation of DNA DSBs, the dCas9-KRAB repressed both pseudo-type VSV.G-HIV-1 NL4-3-ΔE-GFP and wild-type HIV-1 NL43-GFP expression when combined with a gRNA targeting the LTR-R region but not other viral genome sequences ( Supplementary Fig. 4k–m ). It has been known that HIV lentivirus initiates its transcription from the LTR region [31] . Therefore, our result is consistent with a recent study by gRNA library tiling assay that reported the maximum silencing activity of dCas9-KRAB on a target gene in the ∼ 50–100 bp region just downstream of the transcription start sites [32] . We speculate that the higher anti-HIV activity of gRNAs against the LTR region might result from the combinatorial effects of constructive and transcriptional disruption compared with gRNA targeting in other regions (for example, constructive or regulatory regions). The present work indicates that the bacterial CRISPR/Cas9 adaptive immune machinery can be adapted into human cells as a novel anti-virus tool. Our data show that CRISPR/Cas9 can functionally target either the viral coding or non-coding regions during either pre-integration or provirus stages. When DSBs are created by CRISPR/Cas9, presumably exonucleases inside host cells could degrade the viral genome near the DSBs, due to a lack of protection from LTR sequence or LTR-binding proteins in the broken ends. Meanwhile, targeting coding regions can directly disable viral genes through mutations, insertions or deletions [33] . In contrast, when targeting non-coding regions (for example, LTR regions in this study), the structural disruption can be induced in a pre-integration stage, whereas the proviral genome excision can also be achieved in the provirus stage. Our results represent the different targeting/disruption strategies and efficiencies in different stages (pre-integration and provirus), and in different targeting sites as well (coding and non-coding regions). In general, targeting the LTR sequence has a higher impact on HIV-1 expression, especially the LTR-R region ( Fig. 3 ). The LTR-R region contains the TAR sequence that is relatively conserved among the HIV-1 subtypes, which could serve as a common target site for anti-viral disruptions [17] , [34] , [35] . This consequence matches the fact that LTR serves as a critical and universal element for lentivirus expressional regulations by the transcriptional machinery from both virus-encoded proteins and the host cells during the HIV infections [36] , [37] . Regardless of the stage or region targeted, our results show a significant reduction of viral expression by Cas9-mediated antiviral immunity. By using a multiplexed CRISPR/Cas9 system, we achieved an elevated level of disruption and excision of pre-integrated proviral genome. Presumably, using CRISPR/Cas9 directed against multiple conserved target sequences simultaneously can minimize the emergent concern of viral variants developing resistance to singly guided CRISPR/Cas9. In addition, inserting the stably expressed CRISPR/Cas9 system into a T-cell line conferred long-term protection against HIV-1 infection. With recent successful developments, gene-editing technologies have shown great promise in anti-HIV therapy for both pre-clinical studies and ongoing clinical trials [38] , [39] , [40] . As our data show, the system could work on physiologically relevant HIV-1 reservoir cell types and we expect that this system can be further exploited to develop alternative antiviral therapies in the future. Cell culture HEK 293A cell line was purchased from Invitrogen (Carlsbad, CA) and maintained in DMEM medium in 10% fetal bovine serum (FBS), 2 mM glutamine, 1% non-essential amino acids, 1% penicillin–streptomycin. 293T cells were engineered to stably express the CD4 and CCR5 receptors, to generate the 293T.CD4.CCR5 cell line, and were maintained in DMEM supplemented with 10% FBS and 2 μg ml −1 puromycin. Sup-T1 cells from James Hoxie and J-Lat cells from Eric Verdin were obtained through the National Institute of Health (NIH) AIDS Reagent Program. Sup-T1 and J-Lat cells were cultured in RPMI-1640 medium with 10% FBS. H1 hPSC line was purchased from WiCell Research and maintained in human embryonic stem cell medium. Primary T cell Human peripheral blood mononuclear cells were obtained by Ficoll density centrifugation from healthy anonymous blood donors by the San Diego Blood Bank. We have registered with the San Diego Blood Bank to obtain these samples. CD4 + T cells were negatively selected using magnetic beads as per manufacturer’s instructions (CD4 + T-cell enrichment kit, Stemcell Technologies). CD4 + T cells were cultured in RPMI 1640 supplemented with 10% FBS, 100 IU penicillin, 100 μg ml −1 streptomycin, 2 mM L -glutamine and 100 units per ml of interleukin (IL)-2 (Sigma, Saint Louis, MO). Cells were stimulated with a 1:1 ratio of anti-CD3 and anti-CD28 beads (Invitrogen), as per the manufacturer’s instructions, and expanded in the presence of 100 U ml −1 of IL-2. Cells were infected by spinoculation at 1,200 g for 1.5 h in multi-well plates. Retrovirus and adenovirus production For lentiviral vector production, EGFP expression plasmid (pEGIP) was purchased from Addgene (29777) [20] . pEGIP plasmid was packaged and purified as a lentiviral vector according to published papers and the vesicular stomatitis virus Env glycoprotein (VSV-G) is typically used [41] . Non-integrated lentivirus was packaged by pLV-HELP-NIL and pLV-iVSV-G (Invivogen, San Diego, CA), according to the manufacturer’s instructions. Retro reporter virus was prepared by pMX-GFP vector with Retrovirus Gag and Pol components. GFP-transducing unit was determined in 293 cells to define infectious vector titres. For HdAdV production, Venus complementary DNA and Venus-expression HdAdV (pHdAdVenus-geo-TK) were kindly provided by Drs A. Miyawaki and K. Mitani [42] , [43] . The HdAdV production, purification and titration were shown in a previous paper [44] HIV-1 reporter virus preparation and infection HIV-1 NL43-GFP was generated from pNL4-3 Nef + IRES eGFP vector [45] . The HIV-1 R5-Ren_Luc (NL4-3 Nef + IRES rLuc) vector encoding renilla luciferase (rLuc) was derived from NL4-3 Nef + IRES eGFP vector by replacement of the EGFP open reading frame with rLuc and a modification on the envelope to R5-tropic (kindly provided by the Chanda laboratory, Sanford-Burnham Medical Institute, La Jolla). Viral stocks were generated by transfection of HEK 293T cells with 8 μg of pNL4.3 luciferase per 10-cm plate using 300 μl of Lipofectamine 2000. Two days after transfection, the supernatants were collected, clarified at 1,500 r.p.m. for 5 min, filtered (0.45 μM), aliquoted and stored at −80 °C. HIV-1 NL43-GFP viral stocks were concentrated using the Lenti-X concentrator, according to manufacturer’s instructions (Clontech) SupT1 (1.5 × 10 5 ) or CD4 + primary human T cells were pre-treated with Cas9/gRNA mixed with 5.5 or 300 ng of HIV-1 NL43-GFP p24 per well on 96-well plates and spinoculated at 1,200 g for 1 h at room temperature. Plates were incubated at 37 °C for 48 h and viral infection was monitored by flow cytometry. For quantitative chemiluminescent infection assays in monocyte/macrophages derived from hPSCs, cells were plated in 96-well plates and infected with either 3.3 or 6.6 ng p24 of HIV-1 R5-Ren_Luc virus for 72 h. Cells were assayed for rLuc activity using the RenillaGlo reagent (Promega, Madison, WI), according to the manufacturer’s instructions. Plasmid design and construction 2A-mCherry fragment was cloned into the hCas9 vector (Addgene, plasmid 41815) [13] . DNA segment for the chimeric crRNA-tracrRNA was sub-cloned from gRNA cloning vector (Addgene, plasmid 41824) into hCas9-2A-mCherry for single vector purpose. PB backbone plasmid (PB514B-2) was purchased from System Biosciences and the hCas9-2A-mCherry with individual gRNA was sub-cloned into it. The PB-hCas9-2A-mCherry was further modified by replacement of cytomegalovirus promoter and mCherry into CAG promoter and dTomato to generate hPSCs stable lines. For the lentiviral-based CRISPR vector, the Cas9 vector was used from the modification of the lentiCRISPR vector (Addgene, plasmid 49535) [45] , [46] with the replacement of puromycin selection gene to dTomato expression gene and cloning individual anti-HIV gRNA into the vector according the protocol from Addgene. pEGIP*35 plasmid (Addgene, plasmid 26776) [20] was used in the GFP correction experiment to test the activities of hCas9-mCh and its derived constructs. pHR-SFFV-dCas9-BFP-KRAB (Addgene, plasmid 46911) [47] was used in the HIV-1 transcriptional repression experiment. gRNA design and off-target assay Scanning GN 19 NGG motifs on HIV-1 genome identified anti-HIV gRNA candidates that fit with the rules for U6 Pol III transcription and the PAM recognition domain of spCas9 (refs 13 , 48 ). To avoid off-target cleavage of the human genome, the anti-HIV gRNA candidates were filtered to remove the high sequence homology within the entire human genome (build GRCh37.72), especially removing the targets with less than three single-nucleotide mismatches or with low-fidelity sequence in the position 1–5 directly 5′ of the requisite NGG PAM of the CRISPR/SpCas9 (ref. 49 ). The top five off-target candidates were picked from the CRISPR design programme ( http://crispr.mit.edu ) and cloned the flanking ∼ 500 bp from the genomic DNA of anti-HIV CRISPR/Cas9 stable hPSCs or 293 cells for TA cloning and DNA sequencing. The off-target candidates and primer sequences are listed in Supplementary Table 3 . p24 western blotting and ELISA Western blot analysis . Forty-eight hours post infection of 293T.CD4.CCR5 cells with the HIV-1 NL43-GFP virus, 100 μl of supernatant per well was harvested and mixed with 50 μl of 3 × LDS loading buffer. The samples were boiled, separated by SDS–PAGE, transferred to a polyvinylidene difluoride membrane (Millipore) and blotted with a 1:1,000 diluted mouse monoclonal antibody against HIV p24 (0.1 μg μl −1 concentration, MP Cappel, 0856980). The blots were washed, treated with a secondary anti-mouse Alexa 680 nm conjugate (Molecular Probes) and imaged using a LI-COR Odyssey Imager. Full western blot images are shown in Supplementary Fig. 5 . p24 ELISA . The HIV p24 concentration of the viral stocks was measured by p24 antigen capture ELISA, according to manufacturer’s instructions (Zeptometrix). Cas9 western blotting Five hundred thousand cells of H1 hPSC lines with stable expression of Cas9 and anti-HIV gRNA were harvested as pellets and resuspended in 1 × SDS sample buffer. The samples were boiled and separated by 10% SDS–PAGE, transferred to a polyvinylidene difluoride membrane and blotted with 1:1,000 anti-Cas9 monoclonal antibody (Diagenode) or control anti-β-actin (C4) monoclonal antibody (Santa Cruz) at 4 °C overnight. After washing, the blot was treated with a secondary horseradish peroxidase-conjugated anti-mouse IgG (1:5,000, Cell Signaling Technology), reacted in Pierce ECL reagents (Thermo Scientific) and finally exposed to X-ray film for detections. Full western blot images are shown in Supplementary Fig. 5 . Fluorescence microscopy Images of live cells were captured under an Olympus IX51 inverted microscope and analysed using the PictureFrame software. For confocal microscopy analysis, cells were seeded onto Lab-Tek II chamber slides (Thermo Scientific) pre-coated with 0.1% gelatin. After treatments as indicated, cells were then fixed with 4% paraformaldehyde for 30 min at room temperature and washed three times with PBS. Cell nuclei were counter stained with DAPI (4',6-diamidino-2-phenylindole; 1 μg ml −1 , Sigma-Aldrich). Images were captured using a Zeiss LSM780 confocal microscope and were analysed using the ZEN 2011 software. Flow cytometry Cells were collected using TrypLE Express (Life Technologies) and washed twice in PBS with 5% FBS and 2 mM EDTA. Cells were then resuspended in 1 ml PBS with 2 mM EDTA and stained with DAPI (1 μg ml −1 , Sigma-Aldrich), to determine cell viability. Data were acquired on a BD LSRFortessa cell analyser (Becton-Dickinson) and were further analysed using FlowJo software. For single-cell sorting, cells were collected as described above and sorted on a FACSAria II cell sorter (Becton-Dickinson). EGFP- or mCherry-positive cells of desired fluorescence intensity were isolated into 96-well plates preloaded with culture medium with a single cell per well. Provirus copy number detection Copy number detection of Lenti-EGFP and Lenti-mCherry provirus in sorted 293 stable cells was performed following the procedures described in the Lenti-X Provirus Quantitation Kit User Manual from Clontech, with some modifications. Briefly, genomic DNA was extracted from cells using DNeasy Blood and Tissue Kit (Qiagen), according to manufacturer’s instructions. pEGIP and pmCherry vectors for generation of Lenti-EGFP and Lenti-mCherry constructs were used as control templates for the quantitation of Lenti-EGFP and Lenti-mCherry provirus, respectively. The primer sequences for quantitative PCR (qPCR) amplification of provirus were as follows: EGFP forward 5′- ACGACGGCAACTACAAGACC -3′, EGFP reverse 5′- TTGTACTCCAGCTTGTGCCC -3′; mCherry forward 5′- GCGCCTACAACGTCAACATC -3′, mCherry reverse 5′- GCGTTCGTACTGTTCCACGA -3′. qPCR was performed using the SsoAdvanced SYBR Green Supermix (BIO-RAD) on a CFX384 Touch Real-Time PCR Detection System (BIO-RAD). Data analysis and calculations were performed according to the instructions of Lenti-X Provirus Quantitation Kit User Manual (Clontech). Copy number detection of hCas9-mCh-gRNA vector insertion in sorted 293 stable lines was performed similarly as described above, using pmCherry as the control template and mCherry primer sequences for qPCR amplification. Cell viability assay Two hundred and ninety-three stable cell lines containing different hCas9-mCh-gRNAs were plated in triplicate in 96-well plates at a density of 8 × 10 3 per well and allowed to adhere for 24 h. Cells were then either infected with VSV.G-HIV-1 NL4-3-ΔE-GFP , or treated with medium with polybrene only as non-infected controls. Cell viability was assessed 72 h after infection using CellTiter 96 AQueous One Solution cell proliferation Assay kit (Promega), as per the manufacturer’s instructions. Briefly, 20 μl of solution reagent was added into each well of samples and incubated for 1 h at 37 °C. The absorbance at 490 nm was then measured using a plate reader. The relative cell viability percentage for each cell line was then calculated as the ratio of average normalized value (blank-subtracted) in the virus-infected group to the non-infected controls. Relative copy number detection Relative copy number detection of Lenti-EGFP provirus in sorted 293 stable cells was performed 14 days after transfection of different hCas9-mCh-gRNA vectors. Genomic DNA was extracted from cells using DNeasy Blood and Tissue Kit (Qiagen), according to the manufacturer’s instructions. The primer sequences to detect Lenti-EGFP DNA were as follows: EGFP forward 5′- TTGATATCGAATTCCTGCAGCCC -3′, EGFP reverse 5′- GGTGCAGATGAACTTCAGGGTC -3′. GAPDH was amplified to normalize the DNA input and the primer sequences were as follows: GAPDH forward 5′- GGACTCATGACCACAGTCCATGCC -3′, GAPDH reverse 5′- TCAGGGATGACCTTGCCCACAG -3′. qPCR was performed using the SsoAdvanced SYBR Green Supermix (BIO-RAD) on a CFX384 Touch Real-Time PCR Detection System (BIO-RAD). Genomic DNA PCR was performed to confirm the excision of the provirus in the human genome. LTR and GAPDH region were amplified by using the following primers (pEGIP-LTR-F1: 5′- GGGTCTCTCTGGTTAGACCAG -3′, pEGFP-LTR-R1: 5′- TGCTAGAGATTTTCCACACTGACTAA -3′) and GAPDH control primer sequences as above, and under the following PCR condition: 98 °C for 30 s, 32 cycles (98 °C for 10 s, 68 °C for 2 min), 68 °C for 5 min. TA cloning and sequence Genomic DNA was purified by using DNeasy kit (Qiagen). LTR locus was amplified by using the following primers (pEGIP-LTR-F1: 5′- gggtctctctggttagaccag -3′, pEGFP-LTR-R1: 5′- tgctagagattttccacactgactaa -3′) and under the PCR condition: 98 °C for 30 s, 32 cycles (98 °C for 10 s, 68 °C for 2 min), 68 °C for 5 min. GFP locus was amplified by using the following primers (pEGIP T1–7 NO.1 forward: 5′- TTGATATCGAATTCCTGCAGCCC -3′, pEGIP T1–7 NO.1 reverse: 5′- GGTGCAGATGAACTTCAGGGTC -3′) and under the following PCR condition: 98 °C for 30 s, 32 cycles (98 °C for 10 s, 55 °C for 15 s, 68 °C for 20 s), 68 °C for 5 min. PCR products were cloned into pUC118 vector by using Mighty cloning Reagent (TaKaRa) and the independent clones were sequenced. Monocyte/macrophage differentiation from hPSCs The hPSC H1 cell line was used to generate the PB-CRISPR/Cas hPSCs by piggyBac transposon-mediated gene engineering and subsequently differentiated into monocyte/macrophages through spin-EB generation using a feeder-free protocol, which was modified from previous publications [27] , [28] . Cells form spin EBs on 96-well low attachment plates supplemented with cytokines (SCF, VEGF and BMP4) and were grown for 4 days. Medium was changed to StemDiff APEL medium supplemented with cytokines (IL-3 and M-CSF) for 12 days and then removed the IL-3 from the medium for an additional 8 days. An aliquot of cells was analysed using flow cytometry after staining with CD14, CD163, HLA-DR and CD11b, to verify monocyte/macrophage differentiation and the rest of the cells were used for the experiment of HIV-1 R5-Ren_Luc virus challenges. Statistical analysis The statistical analysis represented mean ±s.d. from three or more independent assays. All statistical comparisons were evaluated by unpaired t -test with P -value considered as *** P <0.001; ** P <0.01; * P <0.1; NS, no significant. How to cite this article: Liao, H.-K. et al . Use of the CRISPR/Cas9 system as an intracellular defense against HIV-1 infection in human cells. Nat. Commun. 6:6413 doi: 10.1038/ncomms7413 (2015).